Dynamics of 5-hydroxymethylcytosine during mouse spermatogenesis Little is known about how patterns of DNA methylation change during mammalian spermatogenesis. 5hmC has been recognized as a stable intermediate of DNA demethylation with potential regulatory functions in the mammalian genome. However, its global pattern in germ cells has yet to be addressed. Here, we first conducted absolute quantification of 5hmC in eight consecutive types of mouse spermatogenic cells using liquid chromatography-tandem mass spectrometry, and then mapped its distributions in various genomic regions using our chemical labeling and enrichment method coupled with deep sequencing. We found that 5hmC mapped differentially to and changed dynamically in genomic regions related to expression regulation of protein-coding genes, piRNA precursor genes and repetitive elements. Moreover, 5hmC content correlated with the levels of various transcripts quantified by RNA-seq. These results suggest that the highly ordered alterations of 5hmC in the mouse genome are potentially crucial for the differentiation of spermatogenic cells. To understand how unique epigenetic codes are established is key to elucidate the mechanism of spermatogenesis, a complex developmental process encompassing many cell types including spermatogonia (SG), spermatocytes (SC), spermatids (ST) and spermatozoa (SZ). DNA methylation, one of the best studied epigenetic modifications, is closely related to important biological processes such as X-chromosome inactivation, gene expression regulation, retrotransposon silencing and genomic imprinting [1] , [2] , [3] . Right after germ cell fate is specified, genome-wide DNA demethylation occurs during and after PGC migration [4] , [5] , [6] , [7] , [8] . DNA methylation in germ cells is regained during sex determination. The importance of germ cell DNA remethylation is revealed by the severe phenotypes of DNA methyltransferase-deficient mice [9] . In mice, the majority of methylation in male germ cells is completed before type A SG (SG-A) are formed at 6 days post-partum (dpp), while those at a small number of sites continues to occur until the formation of pachytene SC (pacSC) [10] . Imprinted genes, repetitive sequences and non-promoter intergenic regions complete DNA methylation before birth [9] , [11] , [12] , [13] . However, little is known about whether and how global DNA methylation changes in germ cells after birth. Methylation of cytosine (C) at the fifth carbon position (5mC) has long been regarded as the only stable DNA modification in the mammalian genome until recent discoveries showing that it can be converted to 5-hydroxymethylcytosine (5hmC), 5-formylcytosine (5fC), and 5-carboxylcytosine (5caC) through consecutive oxidation reactions catalyzed by ten-eleven-translocation 1, 2, and 3 (TET1, 2, 3) proteins belonging to the 2OG- and Fe(II)-dependent dioxygenase superfamily [14] , [15] , [16] , [17] , [18] . 5hmC probably exerts regulatory functions as a novel stable epigenetic modification as its content is hundreds-fold higher than 5fC and 5caC in different mouse organs [18] , [19] . Indeed, two recent studies showed that two methyl CpG binding proteins, MeCP2 and Mbd3, preferentially bind to 5hmC and may have important roles in transcription regulation [20] , [21] . Previous studies indicate that 5hmC is enriched in the exons of highly expressed genes in brain tissues, and in cis -regulatory elements such as active enhancers, insulator-binding sites in ESCs [22] , [23] , [24] , [25] , [26] , [27] , [28] . Enrichment of 5hmC is also found in the promoter region of polycomb-repressed ‘poised’ genes in ESCs [23] , [24] , [25] , [27] , which disappeared in the adult brain [29] . By comparing the genomic distribution of 5hmC in mouse hippocampus and cerebellum at three different ages, we have shown that it exhibits dynamic changes during brain development and aging [29] . Here, we use our highly specific 5hmC-labeling and enrichment technique [28] coupled with high-throughput sequencing to profile the global 5hmC distribution in eight germ cell types during spermatogenesis. We analyze the genomic distribution and dynamic changes of 5hmC in genomic regions such as promoters, intra-/intergenic regions of coding and non-coding genes, CpG islands (CGIs), and repetitive sequences during spermatogenesis. Furthermore, we perform RNA-Seq transcriptome analysis at these stages to dissect the functional significance of 5hmC modifications for transcriptional regulation of gene expression. These results provide a genome-wide view of 5hmC profiles during mouse spermatogenesis and reveal the important roles of DNA methylation dynamics in regulating the expression of a large number of genes that drive the progression of spermatogenesis and maintain the identities of spermatogenic cell types. Absolute quantification of 5hmC in mouse spermatogenic cells We isolated eight spermatogenic cell types in the order of their appearance in a single spermatogenic cycle: primitive SG-A (priSG-A), SG-A, type B SG (SG-B), preleptotene SC (plpSC), pacSC, round ST (rST), elongating ST (eST) and SZ. PriSG-A are a mixed population of gonocytes and spermatogonial stem cells, while SG-A are mostly differentiating SG containing a small number of stem cells, and SG-B are differentiated SG ready for meiotic DNA replication. plpSC and pacSC are at the prophase of the first meiotic division. The rest are haploid germ cells ( Fig. 1a ). The purities of these cells were confirmed by morphological evaluation, RT-PCR assessment and immunostaining of well-characterized marker proteins ( Supplementary Fig. S1 , Supplementary Table S1 ). We first determined the absolute levels of 5hmC in these cell types using LS-MS/MS ( Fig. 1b , Supplementary Table S2 ). The percentages of 5hmC relative to C in different germ cells varied by several folds, ranging from 0.03 (rST) to 0.10 (SG-A). It was noteworthy that 5hmC content was the lowest in pacST and rST, two cell types shortly before and after meiosis, and it was higher in diploid germ cells than in haploid ones. In comparison, the Sertoli cells (SE) had higher 5hmC content than male germ cells while mESC had a 5hmC content similar to most germ cells except for rST and eST ( Supplementary Table S2 ). 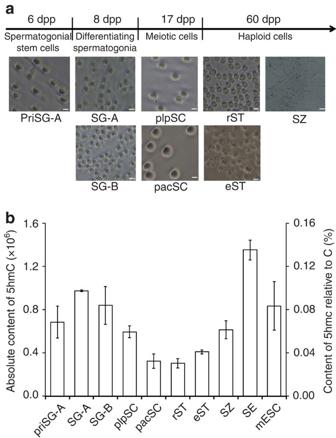Figure 1: Morphological characterization and absolute quantification of 5hmC of mouse spermatogenic cells. (a) Phase contrast photomicrographs of eight isolated spermatogenic cell types. Primitive type A spermatogonia (priSG-A) were isolated from 6 dpp mice; Type A spermatogonia (SG-A) and type B spermatogonia (SG-B) were from 8 dpp mice; preleptotene spermatocytes (plpSC) and pachytene spermatocytes (pacSC) were from 17 dpp mice; and round spermatids (rST), elongating spermatids (eST) and spermatozoa (SZ) were from 60 dpp mice. Scale bar, 10 μm. (b) The absolute levels of 5hmC in eight germ cell types, Sertoli cells (SE) and mESCs are measured as the number of 5hmC in the genome (left-side vertical axis) and the percentages of 5hmC relative to C (right-side vertical axis). The s.e. values of the numbers of 5hmC in the genome are indicated as the error bars. The numbers of samples for priSG-A, SG-A, SG-B, plpSC, pacSC, rST, eST, SZ, SE, and mESC are 2, 3, 3, 5, 3, 4, 5, 3, 3, 3, respectively. The values of 5hmC contents in each cell type and theP-values of pair-wiset-test are detailed inSupplementary Table S2. Figure 1: Morphological characterization and absolute quantification of 5hmC of mouse spermatogenic cells. ( a ) Phase contrast photomicrographs of eight isolated spermatogenic cell types. Primitive type A spermatogonia (priSG-A) were isolated from 6 dpp mice; Type A spermatogonia (SG-A) and type B spermatogonia (SG-B) were from 8 dpp mice; preleptotene spermatocytes (plpSC) and pachytene spermatocytes (pacSC) were from 17 dpp mice; and round spermatids (rST), elongating spermatids (eST) and spermatozoa (SZ) were from 60 dpp mice. Scale bar, 10 μm. ( b ) The absolute levels of 5hmC in eight germ cell types, Sertoli cells (SE) and mESCs are measured as the number of 5hmC in the genome (left-side vertical axis) and the percentages of 5hmC relative to C (right-side vertical axis). The s.e. values of the numbers of 5hmC in the genome are indicated as the error bars. The numbers of samples for priSG-A, SG-A, SG-B, plpSC, pacSC, rST, eST, SZ, SE, and mESC are 2, 3, 3, 5, 3, 4, 5, 3, 3, 3, respectively. The values of 5hmC contents in each cell type and the P -values of pair-wise t -test are detailed in Supplementary Table S2 . Full size image Genomic distribution of 5hmC in mouse spermatogenic cells We applied 5hmC-labeling and enrichment technology coupled with high-throughput sequencing to profile the 5hmC distribution in spermatogenic cells. 5hmC-enriched DNA fragments (also known as reads or tags) were mapped to the mouse genome, and peaks of mapped reads (or hMRs, with an average size of 350 bp) were subsequently identified [30] ( Supplementary Table S3 ). We first examined the 5hmC densities on each chromosome using uni-map reads located in hMRs ( Fig. 2a ). Almost all chromosomes had higher 5hmC content in diploid cells than in haploid ones. The levels of 5hmC correlated positively and significantly with the number of protein-coding genes on each chromosome (Pearson’s r =0.73, P -value=1.61 × 10 −6 , Fig. 2b ). Such a correlation can be visualized by inspecting the abundances of 5hmC and genes on a segment of chromosome 17 ( Fig. 2c ). Similar to brain tissues [29] , the X chromosome was depleted of 5hmC in all types of germ cells ( Fig. 2a ). 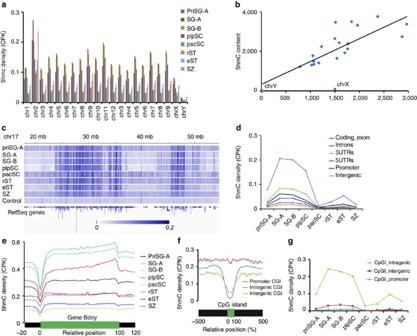Figure 2: Distribution of 5hmC in various genomic regions in eight types of mouse spermatogenic cells. (a) 5hmC densities on the 19 autosomal chromosomes and the X and Y sex chromosomes. (b) The scatter plot of 5hmC levels against the numbers of genes on each chromosome. Note that the point representing the X chromosome is obviously deviated from the fitted line of the plot. (c) Heat map view of 5hmC distribution on a section of chromosome 17 showing that 5hmC level is positively correlated with gene density. (d) Densities of 5hmC (counts per kilobases, CPK) in the hMRs of various genomic regions including promoters (−2 kb to +0.5 kb relative to TSS), exons (5′UTR, 3′UTR, coding-exons), introns, and intergenic regions. (e) 5hmC densities across the gene bodies of all reference genes. (f) 5hmC densities across the CGIs located at the promoter, intragenic and intergenic regions. Only data for priSG-A were shown in this diagram while those for other cell types were shown inSupplementary Fig. S2. (g) 5hmC densities on different types of CGIs for eight mouse spermatogenic cell types. Figure 2: Distribution of 5hmC in various genomic regions in eight types of mouse spermatogenic cells. ( a ) 5hmC densities on the 19 autosomal chromosomes and the X and Y sex chromosomes. ( b ) The scatter plot of 5hmC levels against the numbers of genes on each chromosome. Note that the point representing the X chromosome is obviously deviated from the fitted line of the plot. ( c ) Heat map view of 5hmC distribution on a section of chromosome 17 showing that 5hmC level is positively correlated with gene density. ( d ) Densities of 5hmC (counts per kilobases, CPK) in the hMRs of various genomic regions including promoters (−2 kb to +0.5 kb relative to TSS), exons (5′UTR, 3′UTR, coding-exons), introns, and intergenic regions. ( e ) 5hmC densities across the gene bodies of all reference genes. ( f ) 5hmC densities across the CGIs located at the promoter, intragenic and intergenic regions. Only data for priSG-A were shown in this diagram while those for other cell types were shown in Supplementary Fig. S2 . ( g ) 5hmC densities on different types of CGIs for eight mouse spermatogenic cell types. Full size image Next, we compared 5hmC distributions in various genomic regions. For essentially all cell types analyzed, the level of 5hmC in hMRs was highest on coding exons, followed by 3′UTRs, promoters, introns and 5′UTRs, and was lowest on intergenic regions ( Fig. 2d ). Comparisons with the expected density revealed that 5hmC was enriched in almost all regions except for the intergenic regions and 5′UTRs ( Supplementary Table S4 ). Exons were 5.4–7.1-folds enriched with 5hmC, while intergenic regions were ~40% depleted. Plots of 5hmC tag density within moving windows along the genome indicated that, in all analyzed cell types, the 5hmC level was maintained relatively stably in the gene body of protein-coding genes or increased slightly towards the transcription termination site, and decreased slightly in regions surrounding the gene body on both sides. Moreover, 5hmC was significantly reduced at the transcription start sites (TSSs) ( Fig. 2e ). The density of 5hmC across the genic region was in the order of SG-A, SG-B, plpSC, priSG-A, SZ/eST, rST and pacSC. Finally, we found that 5hmC was depleted in promoter and intergenic CGIs but not in intragenic CGIs ( Fig. 2f , Supplementary Fig. S2a , Supplementary Table S4 ). 5hmC depletion was found in all types of CGIs of high, medium and low GC content, and was positively correlated with GC content ( Supplementary Fig. S2b ). Distribution and dynamics of 5hmC on repetitive sequences We also examined 5hmC distribution on repetitive sequences, which have important roles in spermatogenesis [31] . 5hmC densities were first derived by considering all reads in each type of repeats ( Supplementary Table S4 ). In general, satellite repeats were extremely enriched with 5hmC, several hundreds to a thousand folds enrichments compared with the genome-scale 5hmC density, while the other types of repeats had comparable 5hmC densities with non-repeat genomic regions ( Fig. 3a ). All types of repeats showed a drop from diploid cells to meiotic cells and rST and then an increase in haploid cells. Two deviations from this general pattern were observed. One was that satellites and LINEs reached the lowest level as early as in plpSC with LINEs showing a small surge in pacSC. The other one was that satellites had even higher 5hmC in SZ than in SG-A, which had the highest 5hmC levels in terms of all the other genomic regions ( Fig. 3a ). The 5hmC levels based on uni-map reads located in hMRs showed different dynamic patterns with the densities of 5hmC being much reduced for all types of repeats in all types of cells ( Fig. 3b ). Especially, the 5hmC density in satellites was much less contributed by these uni-map reads, indicating that the overall 5hmC in this type of repeats was mainly contributed by reads mapped to multiple locations. 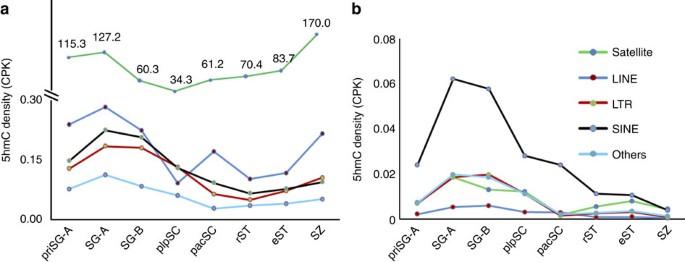Figure 3: 5hmC contents on repetitive sequences. 5hmC densities on different classes of repetitive elements calculated from all reads (a) or uniquely mapped reads (b) exhibited dynamic changes during spermatogenesis. Note that the satellite repeats were prominently enriched with 5hmC (a). Figure 3: 5hmC contents on repetitive sequences. 5hmC densities on different classes of repetitive elements calculated from all reads ( a ) or uniquely mapped reads ( b ) exhibited dynamic changes during spermatogenesis. Note that the satellite repeats were prominently enriched with 5hmC ( a ). Full size image Distribution of dynamic 5hmC regions We then set out to identify hMRs that changed their levels during spermatogenesis, and named them dynamic 5hmC regions (DhMRs) ( Supplementary Table S5 ). The highest numbers of DhMRs were identified during the plpSC/pacSC transition with 109,361 (67.7% of total plpSC hMRs) downregulated. Genomic region enrichment analysis of these DhMRs indicated that they were most enriched in coding exons followed by 3′UTRs, promoters and introns, but were depleted in 5′UTRs and intergenic regions ( Fig. 4a , Supplementary Table S6 ), similar to the genomic distribution of overall hMRs. 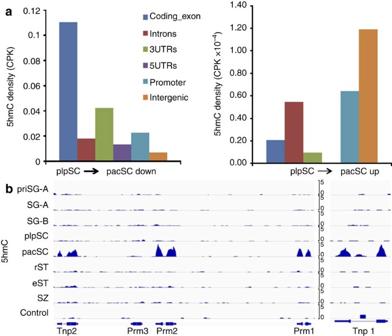Figure 4: Analysis of DhMRs during spermatogenesis. (a) Genomic region distribution of DhMRs downregulated (left panel) or upregulated (right panel) at the plpSC/pacSC transition. (b) An example of pacSC-specific DhMRs located on a cluster of spermatogenic cell-specific genes. Figure 4: Analysis of DhMRs during spermatogenesis. ( a ) Genomic region distribution of DhMRs downregulated (left panel) or upregulated (right panel) at the plpSC/pacSC transition. ( b ) An example of pacSC-specific DhMRs located on a cluster of spermatogenic cell-specific genes. Full size image Interestingly, the corresponding 12,628 genes of the 109361 DhMRs were enriched with functional annotation terms (FATs) related to phosphate metabolism such as ‘phosphate metabolic process’, ‘phosphorus metabolic process’, ‘protein amino acid phosphorylation’ ( Supplementary Tables S5 , Supplementary Data 1 ). The same set of FATs were also enriched in the downregulated DhMRs at the SG-B/plpSC transition, the upregulated DhMRs at the rST/eST transition and the downregulated ones at the eST/SZ transition. Many protein kinase related to these three FATs can be identified at these four transitions. The upregulated DhMRs at the priSG-A/SG-A transition and the downregulated ones at pacSC/rST shared top three FATs ‘regulation of small GTPase-mediated signal transduction’, ‘regulation of Ras protein signal transduction’ and ‘regulation of Rho protein signal transduction’. The upregulated DhMRs at the pacSC/rST transition and the upregulated ones at eST/SZ were enriched with FATs related to RNA transcription and metabolism such as ‘transcription’, ‘regulation of transcription from RNA polymerase II promoter’, ‘regulation of transcription’, ‘metal ion transportregulation of transcription’ and ‘regulation of RNA metabolic process’. Twenty-four transcription factor were in both sets. Moreover, the upregulated DhMRs were identified at the plpSC/pacSC transition and were enriched with ‘gamete generation’, ‘multicellular organism reproduction’ and ‘reproductive process in a multicellular organism’. Well-known post-meiotic germ cell-specific genes were observed in this set, including Smcp , Rnf17, Crem, Spag6, Prm2, Prm1, Tlk2 , Spata16, Adam18 , and so on. The DhMRs located in some genes were indicated by Fig. 4b and Supplementary Fig. S3 . It seemed that DhMRs were closely associated with the expression of germ cell-specific genes. Profiling the transcriptome during mouse spermatogenesis To assess the potential function of 5hmC in gene expression regulation, we profiled RNA expression by RNA-Seq in seven germ cell types ( Supplementary Data 2 ). We previously identified ~3,000 intergenic piRNA clusters in the mouse genome based on small RNA sequencing data [32] . We found that a significant amount of RNA-seq reads in the present study mapped to these piRNA clusters, and we will refer to these genomic regions as predicted piRNA precursor (PPP) genes. Total reads from all cell types mapped to 17,146 protein-coding genes, 1,301 non-coding RNA genes, 1,283 PPP genes and 2,760 other potential genes ( Fig. 5a ). The accuracy of our RNA profiling was confirmed by the agreement of our data with reported expression patterns of a variety of known germ cell marker genes including Dnmt3a ( [33] ), Sycp2 ( [34] ) and Prm1 ( [35] ) ( Fig. 5b , Supplementary Fig. S4 ). Based on our transcriptome data, we also found that Tet1 , 2 and 3 were all expressed at higher levels in diploid germ cells compared with haploid cell types with Tet3 being much more abundant than the other two ( Fig. 5b ). 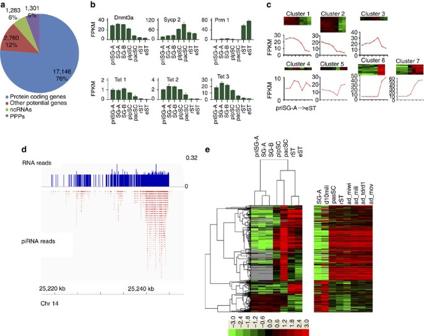Figure 5: Transcriptome profiling of germ cells via RNA-Seq. (a) Classes of different types of genes whose transcripts were identified by RNA-Seq. PPP genes, predicted piRNA precursor genes. (b) Expression patterns of representative marker genes in germ cells as determined by RNA-seq. Theyaxis scales are expression levels in terms of fragments per kb of transcript per million mapped reads. Error bars represents the s.e. determined from duplicate experiments. Note thatTet3is highly expressed in the pre-meiotic cell stages during spermatogenesis. (c) Seven hierarchical clusters (upper panels) were identified based on gene expression patterns during spermatogenesis and their averaged expression levels were shown in the corresponding lower panels. (d) The RNA and piRNA expression of a representative PPP gene in pacSC. Blue and red lines indicate aligned reads from RNA-Seq and piRNA-Seq32, respectively. (e) Heat maps derived from cluster analysis of PPP genes based on RNA-Seq data in this study (left panel) and piRNA-Seq data from previous studies (right panel), of which SG-A, pacSC and rST data were from the study of Ganet al.32, d10 mili data from the study of Aravinet al.52, ad_mili and ad_miwi data from the study of Robineet al.53, ad_tdrd1 data from the study of Reuteret al.54and ad_mov data from Zhenget al.55. D10 mili indicates piRNAs obtained from 10 dpp mouse testis by immunoprecipitation using an anti-MILI antibody. ad_mili, ad_miwi, ad_tdrd1 and ad_mov indicate piRNAs obtained from adult mouse testis by immunoprecipitation using antibodies for MILI, MIWI, TDRD1 and MOV10L1, respectively. Figure 5: Transcriptome profiling of germ cells via RNA-Seq. ( a ) Classes of different types of genes whose transcripts were identified by RNA-Seq. PPP genes, predicted piRNA precursor genes. ( b ) Expression patterns of representative marker genes in germ cells as determined by RNA-seq. The y axis scales are expression levels in terms of fragments per kb of transcript per million mapped reads. Error bars represents the s.e. determined from duplicate experiments. Note that Tet3 is highly expressed in the pre-meiotic cell stages during spermatogenesis. ( c ) Seven hierarchical clusters (upper panels) were identified based on gene expression patterns during spermatogenesis and their averaged expression levels were shown in the corresponding lower panels. ( d ) The RNA and piRNA expression of a representative PPP gene in pacSC. Blue and red lines indicate aligned reads from RNA-Seq and piRNA-Seq [32] , respectively. ( e ) Heat maps derived from cluster analysis of PPP genes based on RNA-Seq data in this study (left panel) and piRNA-Seq data from previous studies (right panel), of which SG-A, pacSC and rST data were from the study of Gan et al. [32] , d10 mili data from the study of Aravin et al. [52] , ad_mili and ad_miwi data from the study of Robine et al. [53] , ad_tdrd1 data from the study of Reuter et al. [54] and ad_mov data from Zheng et al. [55] . D10 mili indicates piRNAs obtained from 10 dpp mouse testis by immunoprecipitation using an anti-MILI antibody. ad_mili, ad_miwi, ad_tdrd1 and ad_mov indicate piRNAs obtained from adult mouse testis by immunoprecipitation using antibodies for MILI, MIWI, TDRD1 and MOV10L1, respectively. Full size image Genes differentially expressed between two adjacent germ cell types were identified using the Cuffdiff package [36] and the most dramatic changes were observed at the transition from plpSC to pacSC, and from pacSC to rST for all four categories of genes listed above ( Supplementary Table S7 ). Hierarchical clustering divided these genes into pre-meiotic and post-meiotic clades, which can further be divided into seven clusters ( Fig. 5c ). The gene expression pattern of each clade/cluster matched well with their function, as suggested by the enriched FATs ( Supplementary Table S8 ). For example, the genes highly expressed pre-meiotically were mainly involved in growth, development, signal transduction, chromatin organization and DNA metabolism, whereas those highly expressed post-meiotically were mainly involved in spermatozoon activity and fertilization. We found that the expression levels of PPP genes closely mirrored the respective piRNA levels ( Fig. 5d ), in agreement with our previous observation [32] . Correlation between 5hmC contents and transcript levels We next determined whether the 5hmC level correlated with gene expression at the mRNA level. In all cell types, genes that contained hMRs in genic or proximal promoter regions were expressed at significantly higher levels than those without hMRs ( Fig. 6a ). Given that the correlation between 5hmC and gene expression may not be linear, we evaluated the correlation by using the Spearman’s Rho correlation coefficient, which ranged from 0.3–0.6 for the seven germ cell types ( Supplementary Table S9 ). Correspondingly, the 5hmC levels on the gene bodies and proximal promoters of highly expressed genes were markedly higher than those of genes expressed at lower levels ( Supplementary Fig. S5a ). We also found that highly expressed genes had lower 5hmC at TSSs than lowly expressed ones ( Supplementary Fig. S5b ). 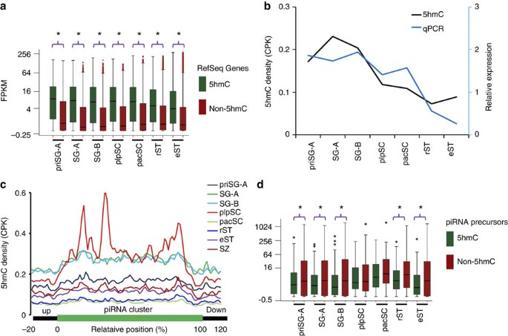Figure 6: Correlation between 5hmC and gene expression during spermatogenesis. (a) Box plots of the expression value of RefSeq genes with (green) or without (red) hMRs in the gene bodies. The expression levels of all RefSeq genes with 5hmC are significantly higher than those without this modification. (b) Positive correlation between expression and 5hmC density of retrotransposons during spermatogenesis. The red line and the left-side vertical axis showed the average levels of 5hmC on all retrotransposons, while the blue line and right-side vertical axis showed the average levels of retrotransposon RNAs. (c) 5hmC densities across the gene bodies of the PPP genes. (d) Box plots of the expression value of PPP genes with (green) or without (red) hMRs in the gene bodies. The expression levels of PPP genes with 5hmC are significantly lower than those without this modification for cell types marked by ‘*’. ‘*’ indicates significant differences based ont-test withP<0.01. Figure 6: Correlation between 5hmC and gene expression during spermatogenesis. ( a ) Box plots of the expression value of RefSeq genes with (green) or without (red) hMRs in the gene bodies. The expression levels of all RefSeq genes with 5hmC are significantly higher than those without this modification. ( b ) Positive correlation between expression and 5hmC density of retrotransposons during spermatogenesis. The red line and the left-side vertical axis showed the average levels of 5hmC on all retrotransposons, while the blue line and right-side vertical axis showed the average levels of retrotransposon RNAs. ( c ) 5hmC densities across the gene bodies of the PPP genes. ( d ) Box plots of the expression value of PPP genes with (green) or without (red) hMRs in the gene bodies. The expression levels of PPP genes with 5hmC are significantly lower than those without this modification for cell types marked by ‘*’. ‘*’ indicates significant differences based on t -test with P <0.01. Full size image We also analyzed the expression of five retrotransposons (LINE-1, MERVL, ORR1, SINE-B1 and SINE-B2) based on their RNA-seq fragments per kb of transcript per million mapped reads values and on qRT-PCR results using separate samples ( Supplementary Fig. S6 ). LINE-1 expression increased from priSG-A all the way to pacSC as indicated by results of both RNA-seq and qRT-PCR, then it continued to increase in rST and eST as shown by RNA-seq data but dropped to a lower level by the qRT-PCR results. The expression of two LTRs (MERVL and ORR1) were both higher before meiosis than after meiosis by two quantitative methods. The expression of the two SINE subfamily members (SINE-B1 and SINE-B2) were consistently identified by both methods, and both decreased their levels from priSG-A all the way to eST. We reasoned that the qRT-PCR results were more accurate than RNA-seq data because more samples and more reliable normalization method were used for the former than for the latter. We plotted the average qRT-PCR expression levels of these five retrotransposons against the average 5hmC densities of LINEs, LTRs and SINEs in the seven spermatogenic cell types. It turned out that the Pearson correlation coefficient ( r ) was 0.79 ( P =0.03) indicating a positive correlation between 5hmC content and the expression of retrotransposons ( Fig. 6b ). We determined the correlation between 5hmC and the transcripts of PPP genes. Interestingly, the enrichment of 5hmC in the genic regions of PPP genes was only apparent in plpSC ( Fig. 6c ). In contrast to protein-coding genes, negative correlations between the expression of PPP genes and their genic 5hmC level were observed for each cell type ( Supplementary Table S9 ). Given that intergenic piRNAs are mainly produced from the pacSC stage onwards [32] , the detection of 5hmC in plpSC suggested that 5hmC might be a precondition for the activation of PPP transcription. Indeed, we found a weak but significant positive correlation between the increase in 5hmC level at SG-B/plpSC transition and the increase in RNA level at the plpSC/pacSC transition ( r =0.2, P =3.6 × 10 −12 ) ( Fig. 6d ). Colocalization of DhMRs with regulatory elements We examined how 5hmC distributed in transcription regulatory sequences, which include proximal promoters, enhancers, insulators marked by epigenetic modifications and/or bound by transcription factors. Shen et al . [37] identified promoter sequences marked by H3K4me3 or bound by polII, enhancers marked by H3K4me1 and H3K27ac, and insulators bound by CTCF in mouse testis. Using SG-A as an example, 5hmC was significantly depleted around the POLII and H3K4me3 peaks in the proximal promoters ( Fig. 7a ). In contrast, it was enriched in non-promoter sequences marked by POLII and H3K4me3. 5hmC was also enriched in enhancers of intergenic and intragenic regions, particularly enhancers marked by H3K4me1. For sequences marked by H3K27ac or H3K27me3, depletion was consistently observed in promoter regions but not in intergenic or intragenic ones. Sequences marked by H3K36me3, which associates with transcription elongation, was enriched with 5hmC. Moreover, CTCF-bound sequences were also depleted of 5hmC at promoters but were enriched with it at intragenic regions. We also checked the overall dynamic changes of 5hmC in these regulatory sequences without distinguishing promoter and non-promoter regions during spermatogenesis ( Fig. 7b ). While the enrichment or depletion of 5hmC in these regulatory sequences basically kept the similar patterns during spermatogenesis, their amplitude varied among cell types. pacSC revealed neither enrichment nor depletion, and SZ possessed the smallest enrichment or depletion if any. The common feature of these two cell types is that their chromatins are highly condensed and the transcription activities are either very low or completely ceased. 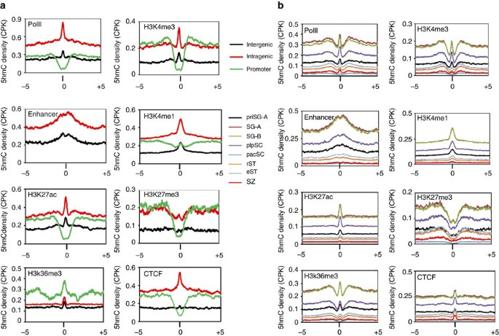Figure 7: 5hmC contents at the regulatory sequences with various chromatin modifications or DNA-binding proteins. (a) 5hmC densities across regions with various chromatin modifications, Pol II and CTCF binding sites located at the promoter (green), the intragenic (red) and the intergenic (black) regions in SG-A cells. (b) The 5hmC contents at different regulatory sequences in eight germ cell types. For each type of regulatory sequences, regions spanning from −5 to 5 kb centering the peak summits were scanned with a moving window to derive the 5hmC densities. The size of the window is 100 bp, and the moving step is 20 bp. Reads located in hMRs were used to calculate 5hmC densities. Figure 7: 5hmC contents at the regulatory sequences with various chromatin modifications or DNA-binding proteins. ( a ) 5hmC densities across regions with various chromatin modifications, Pol II and CTCF binding sites located at the promoter (green), the intragenic (red) and the intergenic (black) regions in SG-A cells. ( b ) The 5hmC contents at different regulatory sequences in eight germ cell types. For each type of regulatory sequences, regions spanning from −5 to 5 kb centering the peak summits were scanned with a moving window to derive the 5hmC densities. The size of the window is 100 bp, and the moving step is 20 bp. Reads located in hMRs were used to calculate 5hmC densities. Full size image We checked whether the DhMR sets possessed any common and specific sequence features by using the MEME software [38] . Interestingly, CT-rich motifs similar to those identified in the mouse brain DhMRs ( [29] ) were also identified in our study ( Supplementary Table. S10 ). We used MEME software to identify the most similar transcription factor-binding sites. It is possible that these transcription factors recruit TET proteins to DhMRs, although their mRNA levels may not always match their putative functional requirements. DNA methylation dynamics in germ cells after birth has not been well addressed. Recent studies have suggested that 5hmC, a stable intermediate of the multi-step 5mC demethylation process, has a regulatory role in ESCs and neurons [39] . As a first step to understand its potential functions during spermatogenesis, we first quantify the absolute levels of 5hmC in eight types of spermatogenic cells, and then use a genome-wide 5hmC-labeling/enrichment/sequencing approach to identify the distribution patterns of 5hmC in various genomic regions and their dynamics. Consistent with previous studies of brain tissues and ESCs, we found that 5hmC was enriched in gene bodies and proximal promoters but depleted in intergenic regions and TSS. 5hmC contents on different types of CGIs was context-dependent, being depleted in CGIs located in promoters and intergenic regions but enriched in intragenic ones as has been observed with ESCs [39] , [40] . We also provide evidence for a positive regulatory role of 5hmC in gene activation during spermatogenesis. It has been estimated that 5hmC is relatively abundant in mouse ESCs and neurons [15] , [28] . According to a previous study by Globisch et al . [41] using HPLC-MS, the 5hmC contents in the spinal cord and testis were estimated to be 0.46 and 0.03% of C, respectively. Using a LC-MS/MS method in the present study, we find that 5hmC contents varies among spermatogenic cells with the lowest in pacSC, rST and eST (0.03~0.04%) and the highest in SG-A and SG-B (0.08–0.10%). That the ratio of 5hmC/C in whole testes by Globisch et al . [41] match well with our values in pacSC and rST reflects the fact that the adult testis is dominated by meiotic and post-meiotic cells. It is noteworthy that mESCs have similar levels to most germ cells except for rST and eST. Interestingly, 5mC levels are constant from priSG-A to SZ and are comparable to that in mESCs ( Supplementary Fig. S7 ), again, consistent with what Globisch et al . [41] observed among different tissues including testes. Therefore, 5hmC, which is approximately <2.5% of 5mC in spermatogenic cells, represents a small but dynamic portion of 5mC during spermatogenesis. A previous study examined genome-wide DNA methylation in postnatal male germ cells by using restriction landmark genomic scanning and the results suggested that cytosine methylation only alters in a small proportion of genomic sites, mainly in early meiotic prophase I ( [10] ). In this line, one of the main contributions of our study is that we have identified this small but dynamic proportion. It is believed that demethylation and remethylation of repeats is mostly completed before birth [9] , [11] , [12] , [13] . In the present study, we show that the 5hmC status in repeats keep changing during spermatogenesis even after birth. The overall 5hmC densities on repeats are similar to or even slightly lower than those on non-repeat sequences except for satellites ( Supplementary Table S4 ). It has been reported that 5hmC is enriched in SINEs, LINEs and satellites in ESCs [22] , while it is only enriched in SINEs and LTRs but depleted in LINEs and satellites in the brain [29] . In the present study, we show that 5hmC distribution in repeats has a unique pattern in spermatogenic cells. It is markedly enriched in satellites in all cell types as expected based on the high level DNA methylation previously observed in heterochromatin encompassing a large amount of satellites. Notably, 5hmC content in all types of repeats are mainly contributed by the multi-map reads, the majority of which map to satellites. Interestingly, the 5hmC dynamics of SINEs described in our study mirror the change pattern of its 5mC precursor reported by Ichiyanagi et al . [42] with higher levels in spermatogonia but lower levels in meiotic and post-meiotic cells. In pacSC, 5hmC is mainly located in LINEs compared with the other types of retrotransposons, in line with the results in a previous study showing that LINE expression can be detected in this cell type [43] . Currently, we do not know why global 5hmC in SZ is higher than pacSC and the other haploid cells, but this observation is consistent with the marked retrotransposon demethylation observed in zygotes shortly after fertilization [44] . The three Tet enzymes that are responsible for the 5mC/5hmC conversion exhibit greater expression in diploid cells than in haploid ones. These expression patterns correlate well with the total levels of 5hmC in the corresponding cell types. For example, these enzymes are expressed at the highest levels in SG-A and SG-B, matching the highest levels of 5hmC in these two cell types. The levels of the enzymes drop precipitously in pacSC, while that of 5hmC also drop significantly. Tet1 and Tet2 were expressed at much lower level than Tet3 in all cell types. Therefore, it is likely that Tet3 is the key enzyme for the production of 5hmC from 5mC in male germ cells as is the case in oocytes and zygotes [45] . Several lines of evidence in the present study support a positive role of 5hmC in gene activation. First, 5hmC levels and the numbers of genes in each chromosome are positively correlated. Second, positive correlations between the levels of 5hmC and various transcripts (mRNAs, retrotransposons and PPPs) are observed. Third, 5hmC reveal unique distributions in different transcription regulatory sequences. Moreover, three spermatogenic cell-specific events supporting the regulatory role of 5hmC are noteworthy. One is related to the highly condensed chromatin states of pacSC and SZ and their consequent global low levels of transcription activity. Correspondingly, the global and regional contents of 5hmC are the lowest in pacSC. Although the 5hmC global content in SZ is medium among all spermatogenic cells, its non-repeat genomic regional contents in SZ are as low as in pacSC. The second special event is the specific expression of a set of protein-coding genes in meiotic and post-meiotic cells. Many such genes, for example, the Tnp2-Prm3–Prm2-–Prm1–Tnp1 cluster, have their 5hmC levels elevated solely in pacSC. The third unique feature of spermatogenic cells is that they produce large amounts of piRNAs that are processed from coding and non-coding RNAs. The presence of 5hmC in the gene bodies of these PPP genes are only observed in plpSC. Therefore, it seems that the elevation of 5hmC in plpSC is a precondition for starting their RNA expression in pacSC. Although the overall genomic distribution of 5hmC, its positive correlation with transcription is obvious, and particular types of genes demonstrating such strong correlation can be identified, it is hard to identify key regulatory sequences that are modified by this novel epigenetic modification. We find that the genomic distributions of 5hmC as well as its correlation with gene expression match well with what people have observed with its precursor 5mC [3] . Therefore, it is possible that the regulatory role of DNA methylation was mediated mainly by 5mC while 5hmC is just a byproduct of a leaky demethylation process. However, several recent studies suggest that 5hmC represents an transcription activating marker recruiting protein partners such as Mbd3/NURD complex and MeCP2 either preferentially or with equal affinity as 5mC [20] , [21] . Therefore, probably 5hmC is the genuine mediator of gene activation although it only occupies a small percentage of 5mC. General description of 5hmC data acquisition F1 mice of DBA/2NCrlVr females and 129S2/SvPasCrlVr males were used for germ cell isolation using the STAPUT method [46] (See Supplementary Methods for details). Ethical clearance was granted by the Research Animal Committee of the Institute of Zoology, Chinese Academy of Sciences. Cells from priSG-A to pacSC were isolated from prepubertal mice undergoing the first wave of spermatogenesis while rST, eST and SZ were from 60 dpp adult mice. The purity of the different cell types all exceeded 85% based on morphological and immunofluorescent evaluations ( Fig. 1 , Supplementary Fig. S1 , Supplementary Table. S1 ). The absolute quantification of 5hmC in various cell types was performed by using LC-MS/MS method. More than 33 million 5hmC-containing DNA fragments (reads) were sequenced for each sample in duplicate and were mapped to the mouse reference genome (mm9) using software Bowtie. Two biological replicates of each cell type, that is, two batches of cells separately isolated from two groups of mice were profiled for 5hmC. To evaluate the reliability of our whole procedure, the correlation of 5hmC levels of the duplicate within 2-kb bins in the genome with 1-kb steps was calculated. The correlation coefficient of each cell type ranged from 0.85–0.98 ( Supplementary Table S3 ), indicating that our 5hmC profiling procedure was highly reliable, as we previously showed [28] , [47] . Reads from the duplicate of each cell type were pooled to identify clusters of reads or otherwise termed peaks or hMRs (5hmC regions) with the MACS software [30] . Among all cell types, ~32–45 million reads were mapped to the genome, covering 57–76% of the 21 million CpGs in the mouse genome, and the average read depth (that is, the number of reads mapped to a CpG) were 2.3–3.3 ( Supplementary Table S3 ). The uniquely mapped reads (uni-map) were ~64–89% of the total mapped reads. Densities for various genomic regions were compared using absolute content-based counts per kilobase (CPK) values. Quantitative analysis of 5hmC in genomic DNA using LC-MS/MS Two micrograms of genomic DNA were digested by nuclease P1 (Sigma), venom phosphodiesterase I (Type VI) (Sigma) and alkaline phosphatase (Sigma). After brief desalting and filter, 10 μl of the solution was injected into LC-MS/MS. The nucleosides were separated by reverse phase ultra-performance liquid chromatography on a C18 column, with online mass spectrometry detection using Agilent 6410 QQQ triple-quadrupole LC mass spectrometer set to multiple reaction monitoring in positive electrospray ionization mode. The nucleosides were quantified using the nucleoside to base ion mass transitions of 258–142 (5hmC) and 228–112 (C). Quantification and detection limits were determined by comparison with the standard curves obtained from nucleoside standards running at the same volume and time. At least two samples of each cell type were used for the quantitative analysis, the original data were shown in Supplementary Table S2 . The abundance of 5hmC (A5hmC) was derived based on the ratio of 5hmC over C (R5hmC/C), the mouse genome size (2.65 × 10 9 bp), the GC content (42%) using the formula: A5 hmC=2.65 × 10 9 × 42% × R5hmC/C ≈10 9 × R5hmC/C ( Fig. 1 ). Chemical labeling of 5hmC and DNA sequencing Genomic DNAs from each cell type were extracted by using Qiagen Blood & Cell Culture DNA Kits following the manufacture’s suggestions and were sonicated into 100–500 bp fragments by using a Covaris S2 instrument. Enrichment of 5hmC-containing DNA fragments was performed followed a procedure detailed in the Supplementary Methods [28] , [29] . Libraries were generated by using Illumina TruSeq Sample Preparation Kits following the manufacturer’s instructions. After PCR amplification, DNA fragments of 250−450 bp were gel-purified and then sequenced by using Illumina Hiseq 2000. 5hmC data processing and analysis Sequenced reads were analyzed using the standard Illumina software. The genomic regions examined included RefSeq protein-coding genes and their 5′UTRs, exons, introns, 3′UTRs, proximal promoters from −2,000 bp to +500 bp relative to the TSS, intergenic regions (complement of protein-coding genes), CGI, repetitive elements represented by RepeatMasker annotated elements. Promoters were classified into three categories based on their CpG content, that is, high, intermediate and low [48] . To compare 5hmC distribution in various genomic regions (g), we calculated the density of 5hmC in a genomic region (Dg) in terms of CPK by using the following formula: Dg=A5hmC × (Rg/Rt)/Lg, in which Rg is the reads mapped uniquely to g and located in hMRs, Rt is the total reads. For repeats, we also used the number of total reads to carry out comparisons. hMRs that demonstrated dynamic changes at the transition from one cell type to the next were termed DhMRs and were identified by using the following algorithm: (1) calculate all fold change values (FCs) of all hMRs between biological duplicates of each cell type; (2) based on the histogram of the FCs, identify the cutoff value of FC so that no more than 5% false positive rate is allowed; (3) calculate hMR intensities (Is) by using formula I =A5hmC × (Rg/Rt) in which g is an hMR; (4) identify all DhMRs based on the above cutoff value and Is. Enrichment analysis of FATs Enrichment analysis of FATs was performed by using the web-based software DAVID and including the Biological Process and Molecular Function Gene Ontology vocabulary. Statistical parameters were such that P <0.01, FDR <0.01 and fold enrichment ≥2. Clustering analysis of the 5hmC level and gene expression Hierarchical clustering of the 5hmC level and gene expression was carried out using the web-based software Cluster ( http://bonsai.hgc.jp/~mdehoon/software/cluster/software.htm#ctv ). Clustering results were visualized with the TreeView program [49] . RNA preparation and sequencing Total RNAs were extracted using QIAGEN RNeasy Mini Kits, and mRNA was isolated by Sera-Mag Oligo (dT) beads (Thermo Scientific) according to the manufacturer’s protocol. Libraries were prepared using the NEB Next mRNA Sample PreP Master Mix Set 1 following the manufacturer’s instructions, and sequenced using Illumina Hiseq 2000. RNA sequence analysis Two biological replicates were profiled for each cell type. The correlation coefficient of transcriptome between the duplicates of the same cell type ranged from 0.95 to 0.99 ( Supplementary Data 1 ), indicating that our RNA-Seq transcriptome data were precise. Again, reads from the duplicate of each stage were pooled for further analysis. The number of reads at each stage ranged from 11–19 million. The sequencing reads were mapped to the mouse genome (mm9) by using the TopHat package [50] . For protein-coding genes and non-coding RNAs, RefSeq genes downloaded from UCSC were used as the reference for assembling transcription units using the Cufflinks software package. The RNA expression level of a gene was represented by fragments per kb of transcript per million mapped reads calculated using the Cufflinks package [36] . For long non-coding RNA(lncRNAs) genes, lncRNAs downloaded from NONCODER (v3, http://www.noncode.org/NONCODERv3/download.htm ) were used as reference. This set was combined with the non-coding RNAs from the Refseq database to give the final non-coding RNA set. PPP genes were defined as genomic regions containing at least 20 intergenic piRNAs with a density of 10 per kb. The differentially expressed genes were identified using the Cuffdiff package. Original data of RNA-Seq in seven cell types during spermatogenesis are included in Supplementary Data 2 . qRT–PCR evaluation of retrotransposon expression Total RNAs were isolated from various cell types using a RNA isolation kit from Tiangen Biotech (Cat. DP420). Two micrograms of RNAs were reversed transcribed in a 30-μl reaction using the Oligo(dT) primer by following the instructions of the Promega Reverse Transcription System (Cat. A3500). The total volume was diluted by four times after the reaction and 1 μl of the solution was used in the subsequent qPCRs conducted on the Roche LightCycler 480 Real-Time PCR system using the UltraSYBR Mixture from Beijing CoWin Biotech (Cat. CW0956). The reaction was set up in the following recipe: 1 μl cDNA template, 7.5 μl 2 × PCR Mix, 0.25 μl forward and reverse primers each (10 μM), 6 μl ddH 2 O. PCR reactions were carried out with a denaturing step (95 °C 10 min) and 45 cycles of denaturing at 95 °C for 15 s followed by annealing and elongation at 60 °C for 1 min. To decide the optimal internal control, we selected 10 genes whose RNA levels keep relatively constant during spermatogenesis based on published microarray data and our RNA-seq data. The top three most stable genes were identified based on our qRT-PCR data from the eight germ cell types using Bioconductor package SLqPCR based on Vandesompele et al method [51] . The geometric mean of Actb, Ubc and Nudcd3 were used as internal control for all qPCR analysis. The delta-Ct values of each gene and the internal control were used to derive the expression of retrotransponsons with the amplification efficient being approximated to be 2 based on the raw data. Sequences of all the primers are listed in Supplementary Table S11 . Accession Codes: the sequence data from this study have been submitted to the NCBI Gene Expression Omnibus under accession number GSE35005 . How to cite this article: Gan, H. et al. Dynamics of 5-hydroxymethylcytosine during mouse spermatogenesis. Nat. Commun. 4:1995 doi: 10.1038/ncomms2995 (2013).